Self-luminescing BRET-FRET near-infrared dots forin vivolymph-node mapping and tumour imaging Strong autofluorescence from living tissues, and the scattering and absorption of short-wavelength light in living tissues, significantly reduce sensitivity of in vivo fluorescence imaging. These issues can be tackled by using imaging probes that emit in the near-infrared wavelength range. Here we describe self-luminescing near-infrared-emitting nanoparticles employing an energy transfer relay that integrates bioluminescence resonance energy transfer and fluorescence resonance energy transfer, enabling in vivo near-infrared imaging without external light excitation. Nanoparticles were 30–40 nm in diameter, contained no toxic metals, exhibited long circulation time and high serum stability, and produced strong near-infrared emission. Using these nanoparticles, we successfully imaged lymphatic networks and vasculature of xenografted tumours in living mice. The self-luminescing feature provided excellent tumour-to-background ratio (>100) for imaging very small tumours (2–3 mm in diameter). Our results demonstrate that these new nanoparticles are well suited to in vivo imaging applications such as lymph-node mapping and cancer imaging. Fluorescence imaging has become a powerful technique to visualize biology in its native physiological settings in a living subject [1] , [2] , [3] , [4] , and has been used even in clinics for guiding surgery in cancer patients [5] . One major obstacle encountered with fluorescence imaging is strong autofluorescence arising from living tissues [6] that significantly compromises imaging sensitivity and specificity. Addressing this technical challenge demands the development of imaging probe s that can emit in the near-infrared (NIR) wavelength range where autofluorescence background is significantly decreased, a spectral window where nanoparticle probes offer great potential. One such example are QD-BRET probes based on bioluminescence resonance energy transfer (BRET) between quantum dots (QD) and a bioluminescent protein R. reniformis luciferase (QD-BRET) [7] , [8] . QD-BRET has been applied to in vitro detection [9] , [10] , [11] , protease and nucleic acid sensing [12] , [13] , [14] and in vivo lymphatic imaging [15] . However, unfavourable in vivo pharmacokinetics of QDs after systemic injection, concerns regarding their in vivo stability and the intrinsic toxicity of heavy metals of the QD nanoparticles have largely limited their applications in translational research [16] , [17] , [18] . In this work, we report the development of new self-luminescing NIR nanoparticles for imaging living mice by integrating BRET and fluorescence resonance energy transfer (FRET) in an energy transfer relay to enable self-luminescing NIR emission. We applied these new nanoparticles to image lymphatic networks of mice and found highly efficient labelling of lymph nodes. Using cyclic arginine-glycine-aspartic (RGD) peptides as the targeting ligand, we demonstrated their high sensitivity for targeted tumour imaging in living mice: a tumour-to-background ratio of over 100 in comparison with a ratio of just 3 to 6 with fluorescence imaging. The self-luminescing NIR NPs offer a more efficient strategy for lymph-node mapping and cancer imaging by combining NIR bioluminescence for in vivo imaging and fluorescence for ex vivo imaging. Preparation of BRET-FRET NIR nanoparticles As outlined in Fig. 1 , a dual resonance energy transfer relay process was used to design self-luminescing NIR nanoparticles by combining BRET and FRET. Semiconductor polymer nanoparticles with poly[2-methoxy-5-((2-ethylhexyl)oxy)- p -phenylenevinylene] (MEH-PPV) as the matrix were used because of their generally low or absent toxicity, bright fluorescence intensity and excellent photostability [19] , [20] , [21] , [22] , [23] , [24] . MEH-PPV NPs absorb maximally at 503 nm ( Fig. 2a ). Luc8 (an eight-mutation variant of R. reniformis luciferase) emits blue light with a peak at 480 nm upon addition of its substrate coelenterazine [25] . The good overlap between the MEH-PPV absorption and Luc8 emission suggests that efficient BRET can occur and generate self-luminescing polymeric nanoparticles. 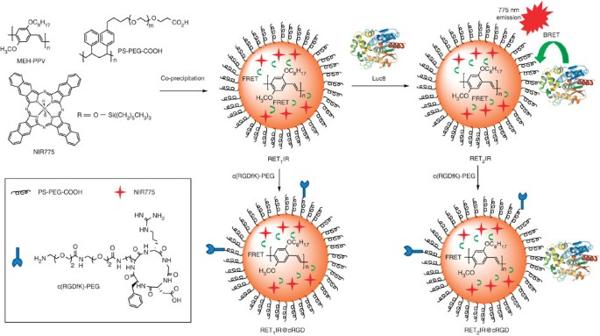Figure 1: Schematic of self-luminescing BRET-FRET NIR polymer nanoparticles. The biochemical energy generated from the Luc8-catalysed oxidation of coelenterazine transfers initially to the MEH-PPV polymer and is then relayed to doped NIR775 dye to produce NIR emission. An amphiphilic polymer, PS-PEG-COOH, coats the nanoparticle to improve water solubility and biocompatibility. Tumour targeting ligands such as cyclic RGD peptides are conjugated to the nanoparticle surface forin vivocancer imaging. Figure 1: Schematic of self-luminescing BRET-FRET NIR polymer nanoparticles. The biochemical energy generated from the Luc8-catalysed oxidation of coelenterazine transfers initially to the MEH-PPV polymer and is then relayed to doped NIR775 dye to produce NIR emission. An amphiphilic polymer, PS-PEG-COOH, coats the nanoparticle to improve water solubility and biocompatibility. Tumour targeting ligands such as cyclic RGD peptides are conjugated to the nanoparticle surface for in vivo cancer imaging. 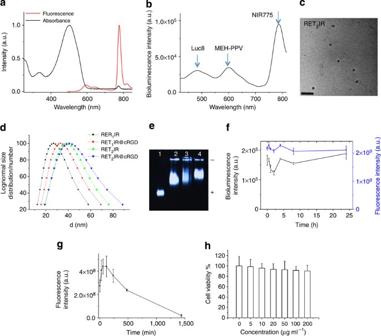Figure 2:In vitrocharacterization of RETIR nanoparticles. (a) Ultraviolet–vis absorption and fluorescence emission spectra ofRET2IRNPs in PBS buffer. (b) Bioluminescence emission spectrum ofRET2IRNPs in PBS buffer. (c) Representative TEM image ofRET2IRNPs. Scale bar=200 nm. (d) Dynamic light scattering (DLS) measurement of four indicated NP formulations in water by lognormal size distribution. (e) Gel electrophoresis (0.5% agarose) analysis of RET NPs in tris-borate-EDTA (TBE) buffer:RET1IR(lane 1),RET1IR@cRGD(lane 2),RET2IR(lane 3),RET2IR@cRGD(lane 4). (f) Bioluminescent and NIR fluorescent intensity ofRET2IRNPs (1 μg) in mouse serum at 37 °C from 0 to 24 h. Data points represent mean±s.d. (n=3). (g) The NIR fluorescence signals of blood samples of mice injected withRET1IRNPs (~20 μg) from 5 min to 24 h. Data represent mean±s.d. (n=4). (h) Viability values (%) of U87MG cells estimated by MTT assay versus incubation concentrations ofRET1IRNPs. Data represent mean+s.d. (n=3). Full size image Figure 2: In vitro characterization of RETIR nanoparticles. ( a ) Ultraviolet–vis absorption and fluorescence emission spectra of RET 2 IR NPs in PBS buffer. ( b ) Bioluminescence emission spectrum of RET 2 IR NPs in PBS buffer. ( c ) Representative TEM image of RET 2 IR NPs. Scale bar=200 nm. ( d ) Dynamic light scattering (DLS) measurement of four indicated NP formulations in water by lognormal size distribution. ( e ) Gel electrophoresis (0.5% agarose) analysis of RET NPs in tris-borate-EDTA (TBE) buffer: RET 1 IR (lane 1), RET 1 IR@cRGD (lane 2), RET 2 IR (lane 3), RET 2 IR@cRGD (lane 4). ( f ) Bioluminescent and NIR fluorescent intensity of RET 2 IR NPs (1 μg) in mouse serum at 37 °C from 0 to 24 h. Data points represent mean±s.d. ( n =3). ( g ) The NIR fluorescence signals of blood samples of mice injected with RET 1 IR NPs (~20 μg) from 5 min to 24 h. Data represent mean±s.d. ( n =4). ( h ) Viability values (%) of U87MG cells estimated by MTT assay versus incubation concentrations of RET 1 IR NPs. Data represent mean+s.d. ( n =3). Full size image To shift the luminescent emission of the nanoparticles to longer wavelengths for in vivo imaging, we doped the polymer matrix with NIR fluorescent dyes such as NIR775 ( Fig. 1 ). Following BRET from Luc8 to the polymer matrix, FRET could occur between the polymer matrix and the doped NIR fluorophore ( Fig. 2a ). This BRET-FRET relay process produces self-luminescing BRET-FRET NIR nanoparticles (abbreviated as RET 2 IR ). Polymer nanoparticles are generally hydrophobic and not water soluble, limiting their biological applications. An amphiphilic polymer, polystyrene graft ethylene oxide functionalized with carboxyl groups (PS-PEG-COOH), was introduced to coat the nanoparticles with a biocompatible shell, orienting its hydrophobic portion within the hydrophobic core of the polymer matrix and exposing its hydrophilic groups towards the nanoparticle surface ( Fig. 1 ). This PEG coating can greatly improve the water solubility and biocompatibility of the nanoparticles, and also help reduce serum protein adsorption and suppress immune reactions, thereby increasing the blood circulation time of the nanoparticles in vivo . The carboxlyate groups presented at the PEG termini are available for bioconjugation of Luc8 and tumour-targeting ligands. RGD peptides have a strong affinity for the cell adhesion receptor integrin α v β 3 , which has a pivotal role in tumour angiogenesis, and have been used for in vivo imaging of a variety of cancers [26] , [27] , [28] , [29] . We conjugated cyclic RGD peptides (cRGD) via their amino groups to the PS-PEG-COOH coated RET 2 IR ( Fig. 1 ) for imaging human glioblastoma U87MG tumour xenografts in nude mice. We first synthesized the MEH-PPV@NIR@PEG nanoparticles (abbreviated as RET 1 IR as there was just FRET in this nanoparticle) using a nanoprecipitation method [30] . To minimize the self-quenching effect among encapsulated NIR dyes, the optimal ratio of NIR775 to the MEH-PPV matrix (by weight) was found to be 0.004–0.02 ( Supplementary Fig. S1 ). Luc8 was conjugated with carbodiimide chemistry between the carboxylate groups on the nanoparticles and the free amino groups on Luc8. The number of Luc8 on each nanoparticle was estimated to be 5.3 on average ( Supplementary Fig. S2 ). The synthesized RET 2 IR NPs were stable in PBS with no aggregation observed after storage at 4 °C at a concentration of 150 μg ml −1 for weeks. Characterization of RETIR nanoparticles The RET 2 IR NPs exhibited a broad ultraviolet/Vis band with a maximum at 503 nm. Under excitation at 490 nm, they exhibited very weak MEH-PPV emission at 594 nm but a strong NIR peak at 778 nm ( Fig. 2a ). At a blending ratio of 0.012 (NIR775/MEH-PPV by weight), the fluorescence quantum yield of the RET 2 IR NPs at 594 nm emission (the polymer matrix) in water dropped from its original value of 0.18 to 0.03 after doping with NIR775, while the quantum yield of the 778 nm emission (NIR775) in water was around 0.09 (in comparison, the quantum yield of free NIR775 in tetrahydrofuran (THF) was 0.08). This result confirms that FRET occurred efficiently from the MEH-PPV matrix to NIR775 in the RET 2 IR NPs. We examined the bioluminescence emission of the RET 2 IR NPs upon addition of coelenterazine. In addition to the emission of Luc8 at 480 nm, two new emission peaks at 594 nm (relatively weak, from MEH-PPV matrix) and 778 nm (strongest, from NIR775) were detected ( Fig. 2b ); this is consistent with our design of the BRET-FRET relay process from Luc8 to the polymer matrix and then to NIR775. The overall BRET ratio, determined by dividing the acceptor emission (550–810 nm) by the donor emission (400–550 nm), was 2.5 (corresponding to an efficiency of 71%), which was nearly double that of QDLuc8 nanoparticles that were previously reported to have a BRET ratio of 1.29 (ref. 7 ). Transmission electron microscopy (TEM) and dynamic light scattering indicated an average particle diameter of ~27 nm for the RET 1 IR NPs ( Fig. 2c ; Supplementary Fig. S3 ). Conjugation to Luc8 and cRGD increased the average hydrodynamic diameter to ~33, 38 and 41 nm for the cRGD conjugated RET 1 IR ( RET 1 IR@cRGD ) NPs, RET 2 IR NPs and the cRGD conjugated RET 2 IR ( RET 2 IR@cRGD ) NPs, respectively ( Fig. 2d ). Gel electrophoresis analysis of these nanoparticles in 0.5% agarose showed a different mobility than the original RET 1 IR NPs because of changes in the surface charge and particle size following bioconjugation ( Fig. 2e ). We examined the stability of the RET 2 IR NPs in mouse serum by monitoring both their bioluminescence and fluorescence at 37 °C for 24 h ( Fig. 2f ). The bioluminescence intensity of nanoparticles remained stable over 24 h and even increased slightly by 10% at 24 h. The fluorescence intensity of the nanoparticles was nearly unchanged with just 3% decrease after 24 h. As expected, the stability of the RET 2 IR NPs in mouse serum was higher at 4 and 22 °C than at 37 °C ( Supplementary Fig. S4 ). In comparison with QDs, the RET 2 IR NPs are more stable in mouse serum and suitable for in vivo imaging applications [16] . The circulation time of the RET 1 IR NPs in the blood was long with an estimated half-life of ~8 h ( Fig. 2g ). The depth of signal penetration of RET 2 IR was assessed both in vitro in a tissue phantom ( Supplementary Fig. S5 ) and in vivo in live mice ( Supplementary Fig. S6 ) in direct comparison with Luc8 and QDLuc8. In the tissue phantom, RET 2 IR luminescence signal was observable even at 2 cm of gel depth at signal intensities significantly greater than QDLuc8, while the signal depth penetration of Luc8 was limited to 1.5 cm ( Supplementary Fig. S5 ). In live mice, the luminescence signal penetration subcutaneously ( Supplementary Fig. S6a,b ) and through the whole animal ( Supplementary Fig. S6c,d ) of RET 2 IR was significantly greater than Luc8, and was equivalent to QDLuc8. In fact an observed advantage of RET 2 IR nanoparticles was the maintained evolution of luminescence signal following the administration of coelenterazine relative to QDLuc8, which exhibited faster signal decay kinetics especially under deeper penetration depths in vivo ( Supplementary Fig. S7 ). The cytotoxicity of the RET 1 IR NPs was evaluated by the methyl thiazolyl tetrazolium (MTT) assay in human glioblastoma U87MG cells, and no significant differences in cell viability were observed in the absence or presence of the RET 1 IR NPs at a concentration of 5–200 μg ml −1 at 37 °C for 24 h ( Fig. 2h ). In conjunction with the imaging depth of penetration studies, these data demonstrate that RET 2 IR nanoparticles are a safer alternative to QDLuc8 as they are free from toxic heavy metals, and that there is no loss of imaging depth penetration performance in vivo . Lymph-node imaging with RETIR nanoparticles At 24 h after tail vein injection of the RET 1 IR NPs into nude mice, the mice were surgically opened for imaging ( Fig. 3a ). Strong NIR fluorescence signals were detected in the lymphatic networks: neck lymph nodes, axillary lymph nodes (AX), lateral thoracic lymph nodes and inguinal lymph nodes (IN) could all be clearly imaged with NIR fluorescence emission. After the removal of internal organs, renal and iliac lymph nodes were also clearly visualized with strong NIR fluorescence ( Supplementary Fig. S8 ). The lymphatic system is difficult to identify because its channels are small and not directly accessible. Nanoparticles have been evaluated for labelling the AX, inguinal lymph node or neck lymph nodes [31] , [32] , [33] , [34] , [35] , [36] . Our results show that the RET 1 IR NPs allow highly efficient labelling of all the lymph nodes in the lymphatic networks after tail-vein injection. 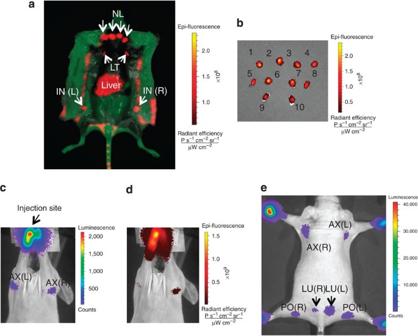Figure 3: Fluorescence and bioluminescence imaging of lymph nodes in mice. (a) Fluorescence imaging of a mouse following and necropsy 24 h after the tail-vein injection ofRET1IRNPs (~20 μg). Superficial skin was removed before imaging but peritoneum was left intact. Autofluorescence is coded in green and NPs signal in red; AX, axillary lymph node; IN, inguinal lymph node; L, left; LT, lateral thoracic lymph node; NL, neck lymph nodes; R, right. (b) Fluorescence image of lymph nodes excised from the mouse in (a): 1–4, NL; 5, AX (left); 6, LT (left); 7, LT (right); 8, AX (right); 9, IN (left), 10 IN (right). (c) Bioluminescence and (d) fluorescence imaging of lymphatic basins in a mouse 10 min after the injection ofRET2IRNPs (~2 μg) intradermally in the forepaws. (e) Bioluminescence imaging of lymphatic basins in a mouse with injection ofRET2IRNPs (~2 μg) intradermally in the forepaws. All bioluminescence images were acquired with 10 s exposure time; L, left; LU, lumbar lymph node; PO, popliteal lymph node; R, right. Figure 3: Fluorescence and bioluminescence imaging of lymph nodes in mice. ( a ) Fluorescence imaging of a mouse following and necropsy 24 h after the tail-vein injection of RET 1 IR NPs (~20 μg). Superficial skin was removed before imaging but peritoneum was left intact. Autofluorescence is coded in green and NPs signal in red; AX, axillary lymph node; IN, inguinal lymph node; L, left; LT, lateral thoracic lymph node; NL, neck lymph nodes; R, right. ( b ) Fluorescence image of lymph nodes excised from the mouse in ( a ): 1–4, NL; 5, AX (left); 6, LT (left); 7, LT (right); 8, AX (right); 9, IN (left), 10 IN (right). ( c ) Bioluminescence and ( d ) fluorescence imaging of lymphatic basins in a mouse 10 min after the injection of RET 2 IR NPs (~2 μg) intradermally in the forepaws. ( e ) Bioluminescence imaging of lymphatic basins in a mouse with injection of RET 2 IR NPs (~2 μg) intradermally in the forepaws. All bioluminescence images were acquired with 10 s exposure time; L, left; LU, lumbar lymph node; PO, popliteal lymph node; R, right. Full size image Similarly, the RET 2 IR NPs (~2 μg) were introduced into the forepaws of mice via intradermal injections. Within 10 min of injection, the AX could be readily visualized non-invasively by bioluminescence imaging ( Fig. 3c ). When followed by in vivo fluorescence imaging, lower fluorescent signals were obtained at the AX in comparison with bioluminescence imaging ( Fig. 3d ). After RET 2 IR NPs were injected into all four paws (each at ~2 μg), all lymph nodes in the same mouse were clearly visualized by bioluminescence imaging ( Fig. 3e ). The axillary and popliteal lymph nodes were still clearly labelled even 10 days later ( Supplementary Fig. S9 ). Tumour imaging with RET 1 IR nanoparticles To evaluate RET 2 IR NPs for cancer imaging, we first tested the cRGD conjugated RET 1 IR ( RET 1 IR@cRGD ) NPs for imaging α v β 3 receptors of human glioblastoma U87MG cells in culture, which express high levels of α v β 3 . After 2.5 h incubation, intense NIR fluorescence was detected at the cell membrane and in the cytoplasm ( Fig. 4a ), of which the cytoplasmic signal increased with time up to 24 h ( Fig. 4b ). DAPI staining revealed little NIR fluorescence signal in the nucleus ( Supplementary Fig. S10 ). In contrast, the control RET 1 IR NPs without cRGD resulted in very weak NIR fluorescence from U87MG cells under the same experimental conditions ( Fig. 4c ). 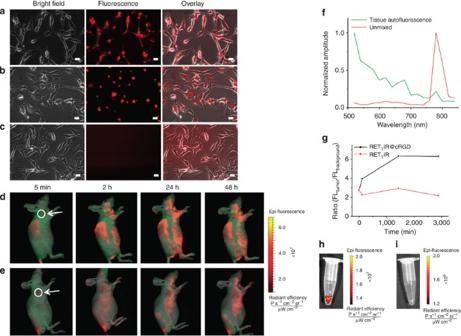Figure 4: Fluorescence imaging of U87MG cellsin vitroandin vivowith RET1IR@cRGD NPs. (a–c) Live imaging of U87MG cellsin vitroincubated withRET1IR@cRGDNPs (4 μg) for (a) 2.5 h and (b) 24 h, or (c) incubated withRET1IRNPs without cRGD for 24 h. Scale bar: 20 μm; excitation: 480/30 nm, dichroic beamsplitter: Q570LP, emission: D755/40M; objective: × 20; acquisition time: 1 s. (d,e) Time-dependent fluorescence imaging of U87MG tumour-bearing mouse (tumours are indicated by white arrows and circles, and are 4 mm in diameter) injected with (d)RET1IR@cRGDor (e)RET1IRNPs (each at ~50 μg) after 5 min, 2, 24 and 48 h. Autofluorescence is coded in green and the unmixed polymer nanoparticle signal in red. (f) Fluorescence spectra of tissue autofluorescence (green) and the unmixed nanoparticle signal (red) in a living mouse. (g) Region of interest (ROI) analysis of fluorescence intensity of tumour over background of mice in (d) and (e). Using one-tailed paired Student’st-test (n=3 mice injected withRET1IR@cRGD),P<0.05 at 24 h. (h,i) NIR fluorescence imaging of urine samples (h) collected 48 h after injection from mouse in (d), and (i) from a mouse without any nanoparticle injection. Figure 4: Fluorescence imaging of U87MG cells in vitro and in vivo with RET 1 IR@cRGD NPs. ( a – c ) Live imaging of U87MG cells in vitro incubated with RET 1 IR@cRGD NPs (4 μg) for ( a ) 2.5 h and ( b ) 24 h, or ( c ) incubated with RET 1 IR NPs without cRGD for 24 h. Scale bar: 20 μm; excitation: 480/30 nm, dichroic beamsplitter: Q570LP, emission: D755/40M; objective: × 20; acquisition time: 1 s. ( d , e ) Time-dependent fluorescence imaging of U87MG tumour-bearing mouse (tumours are indicated by white arrows and circles, and are 4 mm in diameter) injected with ( d ) RET 1 IR@cRGD or ( e ) RET 1 IR NPs (each at ~50 μg) after 5 min, 2, 24 and 48 h. Autofluorescence is coded in green and the unmixed polymer nanoparticle signal in red. ( f ) Fluorescence spectra of tissue autofluorescence (green) and the unmixed nanoparticle signal (red) in a living mouse. ( g ) Region of interest (ROI) analysis of fluorescence intensity of tumour over background of mice in ( d ) and ( e ). Using one-tailed paired Student’s t -test ( n =3 mice injected with RET 1 IR@cRGD ), P <0.05 at 24 h. ( h , i ) NIR fluorescence imaging of urine samples ( h ) collected 48 h after injection from mouse in ( d ), and ( i ) from a mouse without any nanoparticle injection. Full size image The RET 1 IR@cRGD NPs were then injected intravenously into nude mice bearing a U87MG tumour on the left shoulder (~50 μg per animal), and the mice were imaged at multiple time points postinjection ( Fig. 4d ). The in vivo fluorescence spectrum of the RET 1 IR@cRGD NPs was collected from 520 to 840 nm with a bandwidth of 20 nm and an excitation of 465 nm ( Fig. 4f ). As early as 5 min postinjection, enhanced NIR fluorescence signal (780 nm) was observed in the U87MG tumour ( Fig. 4d ), and gradually increased over time. Region of interest measurements showed that the NIR fluorescence signal ratio between the tumour and the surrounding tissue was 2.4±0.6 (5 min), 3.3± 0.7 (2 h), 6.1±0.2 (24 h) and 5.9±0.6 (48 h) ( Fig. 4g ). There was significant fluorescence signal from the skin after 2 h, which complicated the detection of small size tumours, however, the NIR fluorescence signal became stronger when the tumour size became larger, for example, at 8 mm in diameter ( Supplementary Fig. S11 ). In comparison, no significant NIR fluorescence signal was observed in the tumours injected with the non-targeted RET 1 IR NPs ( Fig. 4e ), and the NIR fluorescence signal ratio between the tumour and background was 2.7, 2.2, 2.9 and 2.1 at 5 min, 2, 24 and 48 h, respectively ( Fig. 4g ). The small increase in the NIR fluorescence signal also observed with the non-targeted RET 1 IR NPs is likely due to the enhanced permeability and retention effect. Fluorescence imaging of mice killed 48 h after injection of RET 1 IR@cRGD NPs revealed uptake in the lymph nodes, skin, stomach, bone, liver, spleen and tumour ( Supplementary Fig. S12a, b ). NIR fluorescence signal was also observed in collected urine ( Fig. 4h ), suggesting that RET 1 IR NPs were cleared from the body through the renal system in addition to the hepatobiliary system. Tumour imaging with RET 2 IR nanoparticles The RET 2 IR NPs can emit NIR light in the presence of the substrate of Luc8, coelenterazine, without external excitation and therefore can provide further advantages in comparison with the RET 1 IR NPs. The cRGD conjugated RET 2 IR@cRGD NPs were similarly evaluated in the U87MG tumour xenograft mouse model. After tail vein injection of the RET 2 IR@cRGD NPs, mice were image serially by bioluminescence imaging. At 5 min post injection, strong bioluminescence emission was observed in the U87MG tumour with little signal from other tissues ( Fig. 5a ). The bioluminescence signal ratio between the tumour and background was estimated from region of interest measurements to be 66.0±4.8 (5 min), 116.4±7.6 (2 h), 23.3±16.2 (24 h) and 12.9 (48 h) ( Fig. 5c ). The bioluminescence signal from the U87MG tumour decreased significantly when free cRGD (300 μg) was co-injected intravenously with the RET 2 IR@cRGD NPs ( Supplementary Fig. S13 ), confirming the specific binding of RET 2 IR@cRGD NPs to α v β 3 integrin expressed at the neovascular endothelium of the U87MG tumour. 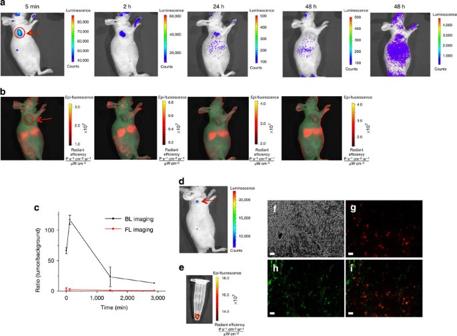Figure 5:In vivoimaging of U87MG tumours in mice with RET2IR@cRGD. (a,b) Time-dependent (a)in vivobioluminescence and (b) fluorescence imaging of U87MG tumour-bearing mouse (indicated by a red arrow and circle; tumour size was about 5 mm in diameter) injected withRET2IR@cRGDNPs (~50 μg). Acquisition time for images in (a) from left to right: 15 s (5 min), 15 s (2 h), 1 min (24 h), 1 min (48 h) and 3 min (48 h). (c) ROI analysis of the bioluminescence and fluorescence intensity between tumour and background of mice in (a) and (b). Using one-tailed paired Student’st-test (n=3),P<0.00002 at 5 min, and 2 h,P<0.04 at 24 h andP>0.05 at 48 h. (d)In vivobioluminescence imaging of a mouse with a small tumour of 2 mm in diameter, as indicated by a red arrow, 2 h after tail vein injection ofRET2IR@cRGD. (e) NIR fluorescence imaging of urine samples collected 48 h after injection from mice in (a). Data points represent mean±s.d. (n=4) (f–i) Histological imaging of frozen U87MG tumour slices from mouse in (a): (f) bright field, (g) NIR fluorescence (excitation filter: 480/30 nm, dichroic beamsplitter: Q570LP, emission filter: D755/40M, acquisition: 1 s), (h) Alexa Fluor 488 anti-mouse CD31 (excitation: 480/30 nm, dichroic beamsplitter: 505DCLP, emission: D535/40 nm, acquisition time: 200 ms) and (i) overlay of images in (g) and (h). Scale bar: 20 μm, objective: × 20. Figure 5: In vivo imaging of U87MG tumours in mice with RET 2 IR@cRGD. ( a , b ) Time-dependent ( a ) in vivo bioluminescence and ( b ) fluorescence imaging of U87MG tumour-bearing mouse (indicated by a red arrow and circle; tumour size was about 5 mm in diameter) injected with RET 2 IR@cRGD NPs (~50 μg). Acquisition time for images in ( a ) from left to right: 15 s (5 min), 15 s (2 h), 1 min (24 h), 1 min (48 h) and 3 min (48 h). ( c ) ROI analysis of the bioluminescence and fluorescence intensity between tumour and background of mice in ( a ) and ( b ). Using one-tailed paired Student’s t -test ( n =3), P <0.00002 at 5 min, and 2 h, P <0.04 at 24 h and P> 0.05 at 48 h. ( d ) In vivo bioluminescence imaging of a mouse with a small tumour of 2 mm in diameter, as indicated by a red arrow, 2 h after tail vein injection of RET 2 IR@cRGD . ( e ) NIR fluorescence imaging of urine samples collected 48 h after injection from mice in ( a ). Data points represent mean±s.d. ( n =4) ( f–i ) Histological imaging of frozen U87MG tumour slices from mouse in ( a ): ( f ) bright field, ( g ) NIR fluorescence (excitation filter: 480/30 nm, dichroic beamsplitter: Q570LP, emission filter: D755/40M, acquisition: 1 s), ( h ) Alexa Fluor 488 anti-mouse CD31 (excitation: 480/30 nm, dichroic beamsplitter: 505DCLP, emission: D535/40 nm, acquisition time: 200 ms) and ( i ) overlay of images in ( g ) and ( h ). Scale bar: 20 μm, objective: × 20. Full size image The RET 2 IR@cRGD NPs allow simultaneous fluorescence and bioluminescence imaging in the same mouse, therefore fluorescence spectral imaging was conducted for comparison. Intense NIR fluorescence signal was observed in the liver, and the NIR fluorescence signal in the tumour was much weaker than the bioluminescence signal ( Fig. 5b ). The fluorescence signal ratio between the tumour and surrounding tissues was 3.4±2.4, 2.4±1.7, 1.3±0.6 and 0.9 at 5 min, 2, 24 and 48 h, respectively ( Fig. 5c ). These results demonstrate that bioluminescence imaging provided much higher sensitivity than fluorescence imaging of tumours in vivo . We further tested the efficiency of the RET 2 IR@cRGD NPs in imaging smaller tumours (tumour size of 2–3 mm in diameter) ( Fig. 5d and Supplementary Fig. S14 ). A strong bioluminescence signal was still observed in the U87MG tumour of the mice at 5 min and 2 h. In comparison, the fluorescence signal in the U87MG tumour was much weaker. These results further demonstrated that bioluminescence showed higher sensitivity than fluorescence in cancer imaging in vivo . In vivo biodistribution of the RET 2 IR@cRGD NPs was similar to that of the RET 1 IR@cRGD NPs except for increased uptake in the lung, which is to be expected owing to the relatively larger size of the RET 2 IR@cRGD NPs ( Supplementary Fig. S15 ). Renal clearance also occurred with the RET 2 IR@cRGD NPs as the NIR fluorescence signal was observed in the urine sample collected at 48 h post injection ( Fig. 5e ). Tumour tissues were excised for sectioning and immunohistochemical staining to confirm the tumour-specific uptake of the RET 2 IR@cRGD NPs ( Fig. 5f–i ). Tumour slices were fixed and stained with vascular endothelium-specific CD31 antibodies to mark tumour blood vessels for 1 h before imaging under a fluorescence microscope. Strong NIR fluorescence was observed within the tumour tissue ( Fig. 5g ), which overlaped well with the green fluorescence signal from the Alexa Fluor 488-conjugated CD31 antibody (Biolegend Inc., San Diego, CA) ( Fig. 5h ). This result suggests the binding of the RET 2 IR@cRGD NPs at the neovascular endothelium of angiogenic tumour blood vessels. Although QDs possess excellent optical properties as an imaging probe, concerns such as unfavourable in vivo pharmacokinetics after systemic administration, their instability in vivo and intrinsic toxicity because of their formation from toxic heavy metals have limited their use for translational research. In comparison, the self-luminescing NIR NPs show high stability in mouse serum and increased circulation time ( Fig. 2f ). Importantly, they do not contain any heavy toxic metals. At a size of around 30–40 nm in diameter, they primarily undergo hepatobiliary clearance in mice, but renal clearance has also been observed ( Figs 4h , 5e ). Combined, all these features make the RET 2 IR nanoparticles highly attractive for in vivo imaging research. An important application of fluorescent nanoparticles is lymph-node mapping and imaging that traditionally uses vital blue dyes and radioactive tracers in clinics [35] . We have shown highly efficient labelling of all lymph nodes in the lymphatic networks of mice after a single tail-vein injection of RET 1 IR NPs. Bioluminescence imaging with RET 2 IR@cRGD NPs gave a tumour-to-background ratio of over 100 and very small subcutaneously implanted tumours (2 or 3 mm in diameter) have been clearly imaged within just 5 min after the tail-vein injection of the RET 2 IR@cRGD NPs. This level of sensitivity is at least an order of magnitude higher than fluorescence imaging. With further optimization, tumours <1 mm in diameter may be readily detectable with the self-luminescing NIR probes. To the best of our knowledge, our RET 2 IR NP is the first demonstration of a BRET-FRET relay process for in vivo imaging. The relay uses a Renilla luciferase mutant as the BRET donor, semiconductor polymer MEH-PPV matrix as both the BRET acceptor and the FRET donor, and an NIR dye as the FRET acceptor. The energy transfer relay process was surprisingly efficient. The BRET-FRET relay strategy now allows the use of fluorescent materials other than QDs in building self-luminescing NIR probes for in vivo imaging as long as proper fluorophores are chosen to relay the excitation energy from Renilla luciferase to the NIR dye dopant, even in multiple relaying steps. Further fine tuning of the probe by matching multiple BRET and FRET pairs should enable self-luminescing NIR NPs for multiplex in vivo imaging [21] . Materials The poly(phenylene vinylene) derivative poly[2-methoxy-5-(2-ethylhexyloxy)-1,4- phenylenevinylene] (MEH-PPV; MW: 200,000 Da; polydispersity, 4.0) were purchased from ADS Dyes, Inc. (Quebec, Canada). PS-PEG-COOH (MW: 21,700 Da of the PS moiety; 1,200 Da of PEG-COOH; polydispersity, 1.25) were purchased from Polymer Source Inc. (Quebec, Canada). Silicon 2,3-naphthalocyanine bis(trihexylsilyloxide) (NIR775) was purchased from Sigma Aldrich, Inc. Cyclic RGD peptide was purchased from Peptides International, Inc. All the other chemicals were purchased from Sigma Aldrich, Inc. and used without purification. Luc8 was prepared according to our previously published procedures [8] . Synthesis of NIR nanoparticles NIR775-doped NIR nanoparticles were prepared using a nanoscale precipitation technique [30] . In a typical procedure, a solution of THF containing 50 μg ml −1 of MEH-PPV, 50 μg ml −1 of PS-PEG-COOH and 0.6 μg ml −1 of NIR775 dye was prepared. An aliquot of the mixture (5 ml) was then quickly dispersed into 10 ml of water under vigorous sonication. Extra THF was evaporated at an elevated temperature (below 90 °C) under the protection of nitrogen. The THF-free NPs solution was filtered through a 0.2-μm cellulose membrane filter. Bioconjugation was carried out by EDC-mediated coupling reaction between the carboxyl groups on the NPs and the amine-containing molecules (Luc8 and RGD peptide). In a typical conjugation reaction, 60 μl of concentrated HEPES buffer (1 M) were added to 3 ml of a solution of the carboxylate-presenting NP (50 μg ml −1 in water) and the amine-containing molecules (100 μl of Luc8 at 3 mg ml −1 and 30 μl of RGD peptide at 10 mg ml −1 ), followed by vortex mixing. Then, 50 μl of freshly prepared aqueous EDC solution (10 mg) was added and the above mixture was magnetically stirred for 1 h at room temperature. The uncoupled free Luc8 and excess EDC were removed by four washes using a 100 K Amicon Ultra filter (Millipore Corporation) under centrifugation at 3,000 r.p.m. for 3 min at 4 °C. The final complex was kept in PBS buffer at 4 °C. In vitro nanoparticles characterization The size and morphology of the nanoparticles were investigated using TEM (FEI Tecnai G2 F20 X-TWIN, 200 kV). TEM samples were prepared by dripping the NP solution onto a carbon-supported copper grid and drying at room temperature before observation. The hydrodynamic size of the nanoparticles was also measured in aqueous solution by dynamic light scattering (Brookhaven 90 plus nanoparticle size analyser). The absorption spectra were recorded on an Agilent 8453 ultraviolet–vis spectrometer. Fluorescence and bioluminescence emission spectra were collected with a FluoroMax-3 (Jobin Yvon Inc.) and corrected for wavelength-dependent detector sensitivity as described by the company. In the case of bioluminescence, the excitation light was blocked. Cell culture, cytotoxicity assay and cell imaging U87MG (human glioblastoma, high α v β 3 expression) cells were grown in DMEM supplemented with 10% FBS. Cultures were maintained at 37 °C under a humidified atmosphere containing 5% CO 2 . Cytotoxicity in the U87MG cell line was measured using a MTT assay. Cells growing in log phase were seeded into a 96-well cell culture plate at 1 × 10 4 cells per well and then incubated for 24 h at 37 °C under 5% CO 2 . RET 1 IR NPs (100 μl per well) were added to the wells of the treatment group at varying concentrations, and 100 μl per well DMEM was added to the negative control group, followed by incubation of the cells for 24 h at 37 °C under 5% CO 2 . Subsequently, 10 μl of MTT (5 mg ml −1 ) was added to each well of the 96 well assay plate and incubated for an additional 4 h at 37 °C under 5% CO 2 . After the addition of DMSO (200 μl per well), the assay plate was allowed to shake at room temperature for 20 min. A Tecan microplate reader was used to measure the OD 570 (absorbance value) of each well with the background subtraction at 690 nm. The following formula was used to calculate the viability of cell growth: cell viability (%)=(mean of absorbance value of treatment group/mean of absorbance value of control) × 100. For cell imaging experiments, 5 × 10 5 cells per well were seeded on 18 mm glass coverslips and cultured for 24 h before imaging with a Zeiss Axiovert 200M Microscope (excitation: 480/30 nm; dichroic beamsplitter: Q570LP; emission: D755/40M; objective: × 20; acquisition time: 1 s). Blood circulation half-life in mice The RET 1 IR NPs (~20 μg) were injected intravenously into the tail veins of three six-week-old nude mice. At various time points postinjection, ~20 μl of blood was collected from the tail into 50 μl of 0.9% NaCl solution containing 1.5 mg ml −1 of EDTA. The NIR fluorescence intensity of blood samples was assayed on an IVIS spectrum imaging system (excitation: 465±15 nm; emission: 780±10 nm). Blood samples without the RET 1 IR NPs were measured to determine the blood autofluorescence level, which was subtracted from the fluorescence intensity of injected samples. Biodistribution studies Mice were killed by cervical dislocation under deep isoflurane anaesthesia. Urine samples were immediately collected, and lymph nodes, brain, spleen, pancreas, kidney, lung, heart, liver, bone (femur), muscle (hind leg), stomach (emptied) and dorsal skin were harvested; for tumour-bearing mice, tumours were also harvested. Tissues were subjected to fluorescence imaging using an IVIS spectrum imaging system immediately (excitation: 465±15 nm; emission: 780±10 nm). Lymph-node imaging Mice were anesthetized with 2.5% isoflurane, and RET 1 IR NPs (~20 μg) were administered to nude mice by tail-vein catheterization using the Vevo MicroMarker TVA (Vascular Access) Cannulation Kit (VisualSonics). The tail vein was further flushed with 100 μl of PBS buffer. At 24 h after injection, mice were killed, dissected to locate the lymph nodes of interest and imaged using an IVIS spectrum imaging system immediately (excitation: 465±15 nm; emission: 780±10 nm). Alternatively,~10 μl of RET 2 IR NPs (~2 μg each) were administered to the forepaws via intradermal injections. Within 10 min of injection, mice received an intravenous injection of 10 μg of coelenterazine for in vivo bioluminescence imaging (acquisition time: 10 s; no emission filter). Following bioluminescence imaging, in vivo fluorescence imaging was carried out (excitation: 465±15 nm; emission: 780±10 nm). Tumour implantation and in vivo imaging Animal procedures were approved by the Institutional Animal Care Use Committee of Stanford University. Tumour cells were harvested by incubation with 0.05% trypsin-EDTA when they reached near confluence. Cells were pelleted by centrifugation and resuspended in sterile PBS. U87MG cells (2 × 10 6 cells per site) were implanted subcutaneously into the left shoulder of 4- to 5-week-old female nude mice (Charles River Breeding Laboratories). When the tumours reached the size of 2–8 mm in diameter (2 to 3 weeks after implantation), the tumour-bearing mice were subjected to biodistribution and imaging studies. In vivo and ex vivo fluorescence imaging was performed with an IVIS spectrum imaging system (excitation: 465±15 nm filter; emission: collected from 520 to 840 nm with a bandwidth of 20 nm). For bioluminescence imaging, the mice were imaged after tail vein injection of coelenterazine (20 μg per mouse in 20 μl of methanol and 80 μl of phosphate buffer). Images were acquired without filters. Histology Tumour-bearing mice were euthanized 48 h after injection with RET 2 IR @ cRGD . Tumour tissues were collected, washed with PBS, frozen by dry ice and stored at −80 °C. Frozen samples were cryosectioned by microtome at −20 °C into slices of 5 μm thickness, and then fixed in cold acetone for 5 min (−20 °C). Nonspecific binding sites were blocked over 30 min with PBS containing 10% mouse serum. The sections were stained with 1 μg of Alexa Fluor 488 anti-mouse CD31 antibody in 100 μl PBS buffer for 1 h at 37 °C. The sections were washed with PBS and analysed under a Zeiss Axiovert 200M Microscope. How to cite this article: Xiong, L. et al. Self-luminescing BRET-FRET near-infrared dots for in vivo lymph-node mapping and tumour imaging. Nat. Commun. 3:1193 doi: 10.1038/ncomms2197 (2012).